High-power lithium ion microbatteries from interdigitated three-dimensional bicontinuous nanoporous electrodes High-performance miniature power sources could enable new microelectronic systems. Here we report lithium ion microbatteries having power densities up to 7.4 mW cm −2 μm −1 , which equals or exceeds that of the best supercapacitors, and which is 2,000 times higher than that of other microbatteries. Our key insight is that the battery microarchitecture can concurrently optimize ion and electron transport for high-power delivery, realized here as a three-dimensional bicontinuous interdigitated microelectrodes. The battery microarchitecture affords trade-offs between power and energy density that result in a high-performance power source, and which is scalable to larger areas. Microelectronics have benefitted from continuous miniaturization and integration, whereas there has been much less progress in miniaturization and integration of power sources [1] . Today, except for capacitors, power sources are connected to electronic devices through wiring and circuit traces. Although capacitors can be integrated into electronics, few capacitors have energy density approaching that of batteries [2] , [3] , [4] . Batteries can store considerably more energy than capacitors, but deliver lower power than capacitors and have proven difficult to miniaturize and integrate. Here we demonstrate a high-power and high-energy density microbattery constructed from interdigitated three-dimensional (3D) bicontinuous nanoporous electrodes. The performance of power sources is typically measured by power and energy stored per unit mass or unit volume. For conventional lithium ion batteries, typical volumetric energy and power densities are around 10–60 μW h cm −2 μm −1 and 1–100 μW cm −2 μm −1 . It is possible to achieve higher power density, up to 1,000 μW cm −2 μm −1 , by using porous battery electrodes that reduce ion diffusion through the active anode and cathode materials, as well as designs that reduce ion diffusion time in the electrolyte and decrease electrical resistance in the electrodes [5] , [6] , [7] , [8] , [9] , [10] , [11] . Most publications on high-power batteries focus on either anode or cathode half cells, and show improved power density at the expense of energy density. In principle, a battery architecture based on 3D integrated porous microelectrodes could achieve high-power density without sacrificing energy density by combining small ion diffusion distances, large percentage of active material and highly conductive electrodes. Such a microarchitecture could also enable miniature batteries suitable for microelectronics integration [12] . Previous research on microbatteries has focused on achieving high areal energy density rather than volumetric energy density or volumetric power density, leading to 3D microbattery energy and power densities 0.01–7 μW h cm −2 μm −1 and 0.04–3.5 μW cm −2 μm −1 ( [13] , [14] , [15] , [16] , [17] ). It has proven difficult for batteries of any size to achieve the high power of a supercapacitor, which can be fabricated at nearly any size and have power density larger than 4.0 mW cm −2 μm −1 (refs >4 , 18 ). It is challenging to integrate 3D electrodes into a complete microbattery cell, owing to the difficulty of integrating 3D elements of anode and cathode materials, along with the need to control materials uniformity and feature sizes across a range of length scales of 10 nm–1 mm. A number of 3D half-cell electrode designs for microbatteries, consisting of only the anode or cathode, have been presented [10] , [13] , [19] , [20] , [21] , [22] , [23] . There are, however, only a few publications reporting the performance of microbattery cells having fully integrated 3D anodes and cathodes [13] , [14] , [15] , [16] . Here we present lithium ion microbatteries with power densities up to 7.4 mW cm −2 μm −1 and energy densities up to 15 μW h cm −2 μm −1 . Our batteries meet or exceed the power densities of the best supercapacitors, while retaining comparable energy density [2] , [3] , [4] . Compared with other 3D microbatteries, our batteries have 2,000 × greater power density and 2 × greater energy density [13] , [14] , [15] , [16] . 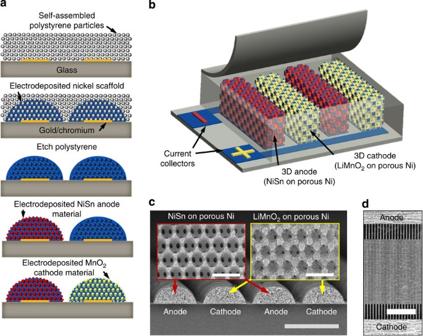Figure 1: Microbattery fabrication and design. (a) Schematic of the fabrication process where the nickel scaffold defines that the battery architecture and the active materials are electrodeposited onto the nickel scaffold for precise integration of the electrodes on a single substrate. (b) Microbattery design. The nanoporous microbattery electrodes consist of an electrolytically active layer (red and yellow) coated on an electrically conductive bicontinuous nickel scaffold (blue). The nickel scaffold acts as the current collector attached to an outside circuit. A nickel–tin alloy is used as the anode (red), and lithiated manganese oxide as the cathode (yellow). (c) Scanning electron microscopy (SEM) cross-section of the interdigitated electrodes spanning two periods. The interdigitated electrodes alternate between anode and cathode. The insets show the magnified electrodes with the nickel scaffold coated with nickel–tin on the left and lithiated manganese oxide on the right. Scale bars, 50 μm and 1 μm in the insets. (d) A top-down SEM image of the interdigitated electrodes with the anode electrodes connecting at the top, cathode electrodes connecting at the bottom and the interdigitated anode and cathode electrodes overlapping in the middle. Scale bar, 500 μm. Microbattery architecture Figure 1 shows the microbattery cell architecture. The electrodes are a thin layer of nickel–tin (anode) or lithiated manganese oxide (LMO) (cathode) conformally coated onto interdigitated highly porous metallic scaffolds. The microarchitecture provides short electron and ion transport lengths in the electrolytically active material and electrolyte (yielding high-power density) while maintaining a high volume of active material (yielding high-energy density) [6] , [24] . The active material thickness varies between 17 and 90 nm. The metallic scaffold has 330- or 500-nm diameter pores. The interdigitated electrodes have a width of 30 μm and spacing of 10 μm, and the full battery cell has a volume of about 0.03 mm 3 . The architecture based on interdigitated porous electrodes allows control over the disparate length scales necessary for high power and overcomes the challenge of fabricating full cells on a single substrate by allowing independent electrodeposition of the active materials onto their respective metallic scaffolds, taking advantage of the anode and cathode electrical isolation. Figure 1a illustrates the fabrication advantage of electrodeposition. We designed eight different batteries (A–H) with variations of pore size, active material thickness and battery geometry ( Supplementary Table S1 ). Figure 1: Microbattery fabrication and design. ( a ) Schematic of the fabrication process where the nickel scaffold defines that the battery architecture and the active materials are electrodeposited onto the nickel scaffold for precise integration of the electrodes on a single substrate. ( b ) Microbattery design. The nanoporous microbattery electrodes consist of an electrolytically active layer (red and yellow) coated on an electrically conductive bicontinuous nickel scaffold (blue). The nickel scaffold acts as the current collector attached to an outside circuit. A nickel–tin alloy is used as the anode (red), and lithiated manganese oxide as the cathode (yellow). ( c ) Scanning electron microscopy (SEM) cross-section of the interdigitated electrodes spanning two periods. The interdigitated electrodes alternate between anode and cathode. The insets show the magnified electrodes with the nickel scaffold coated with nickel–tin on the left and lithiated manganese oxide on the right. Scale bars, 50 μm and 1 μm in the insets. ( d ) A top-down SEM image of the interdigitated electrodes with the anode electrodes connecting at the top, cathode electrodes connecting at the bottom and the interdigitated anode and cathode electrodes overlapping in the middle. Scale bar, 500 μm. Full size image Performance of the microbattery cells Table 1 presents the volumetric energy and average power density of our microbattery cells and also lists the performance characteristics of 3D microbattery cells from the literature. The volume used for the calculations is the entire cell volume, including the volume occupied by the electrodes and between electrodes. At a 1.5-C discharge rate, our microbattery cell A has a 15 μW h cm −2 μm −1 energy density and 23 μW cm −2 μm −1 power density, 2 × the energy density and 6 × the power density of the best published cells [13] , [14] , [15] , [16] . At an 870-C discharge rate, microbattery cell B has a 0.6 μW h cm −2 μm −1 energy density and 7.4 mW cm −2 μm −1 power density, a larger energy density than three of the four published cells and 2,000 × the power density of the best published cell [13] , [14] , [15] , [16] . Supplementary Table S2 shows the energy and power density of microbattery cells A–H. Table 1 Volumetric energy and power density of our microbattery cells (A and B) and published 3D microbattery cells (MB1-MB4). 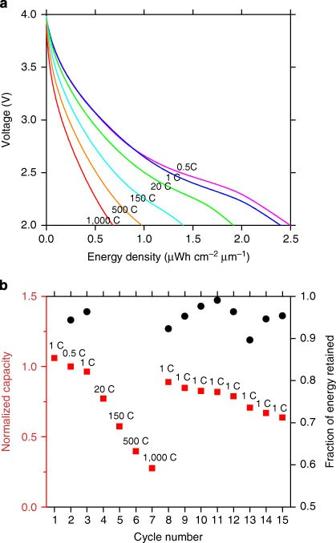Figure 2: Electrochemical properties of the microbattery. (a) Discharge from microbattery cell H at C rates ranging 0.5–1,000. (b) Capacity of microbattery cell H for the first 15 cycles at the noted C rate, normalized to the energy at 0.5 C. The secondaryyaxis indicates the percentage of capacity retained in the given cycle when compared with the previous cycle (calculated for low C rate cycles only). Full size table Figure 2a shows the discharge data of microbattery cell H. At 1 C, the battery is near steady state, because its energy is 96% of its energy at 0.5 C. At high discharge rates, the cell retains a large percentage of its low rate energy, 28% at 965 C. Supplementary Figs S1 and S2 show the discharge of cell H versus time and the discharge of cells A through H. Figure 2b shows the normalized discharge capacity of microbattery cell H after 15 charge/discharge cycles. The microbattery cell retains 92% of its energy after four high rate discharges. The cell retains 64% of its initial energy after 15 cycles, loosing on average 5% of its energy after each low rate cycle. One reason for capacity fade may be the lithium capacity in the anode and cathode were not matched, such that the anode acted as a large ion source but reduced the number of transportable ions because of irreversible capacity loss from SEI formation after each cycle. Figure 2: Electrochemical properties of the microbattery. ( a ) Discharge from microbattery cell H at C rates ranging 0.5–1,000. ( b ) Capacity of microbattery cell H for the first 15 cycles at the noted C rate, normalized to the energy at 0.5 C. The secondary y axis indicates the percentage of capacity retained in the given cycle when compared with the previous cycle (calculated for low C rate cycles only). 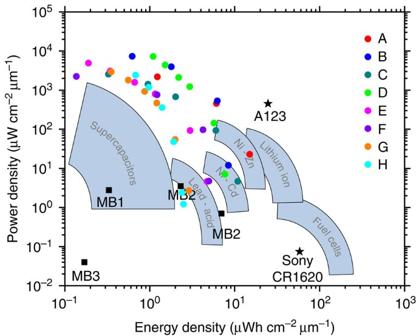Figure 3: Ragone plot showing the performance of our microbattery cells and conventional power technologies. The energy and power density of our microbattery cells (A–H) at low to high C rates, along with previous microbattery cells having 3D electrodes (MB1 through MB3). The plot also includes the performance range of conventional power technologies and commercial batteries from A123 (high power) and Sony (high energy). Full size image Figure 3 presents a Ragone plot of the energy and power densities of microbattery cells presented here, along with conventional energy-storage technologies including two commercial batteries. The energy densities of our microbattery cells at low rates vary from 2.5 to 15 μW h cm −2 μm −1 . At high rate (order of 1000 C), our microbatteries have power densities up to 7400 μW cm −2 μm −1 . Compared with conventional supercapacitors, our microbattery delivers 10 × the power of a supercapacitor at comparable energy density, delivers 10 × the energy of a supercapacitor at comparable power density or has 10 × smaller volume than a supercapacitor at comparable performance. Supplementary Fig. S3 and Supplementary Note 1 provide further comparison with supercapacitors. Figure 3: Ragone plot showing the performance of our microbattery cells and conventional power technologies. The energy and power density of our microbattery cells (A–H) at low to high C rates, along with previous microbattery cells having 3D electrodes (MB1 through MB3). The plot also includes the performance range of conventional power technologies and commercial batteries from A123 (high power) and Sony (high energy). Full size image The microbattery architecture reported here improves power density and enables microelectronics integration of lithium ion batteries. The high-power density is achieved by simultaneously reducing ion diffusion lengths and electrical resistances across the entire microbattery system. The architecture allows compact integration of the anode and cathode on a single substrate for microelectronics applications. This work illustrates how a micro-engineered architecture and material integration can improve performance and enable the integration of miniature power sources, which have broad applications from medical implants to remote sensor networks. The batteries could be further improved by taller 3D electrodes, which would require improvements in the fabrication process. Additional research could explore the fundamentals of ion transport in this type of 3D battery, explore other battery chemistries and routes to microelectronics packaging. Nickel scaffold and microbattery architecture fabrication We fabricated the fully integrated microbattery cells with anode, cathode and liquid electrolyte by growing 3D porous electrodes on electrically isolated, interdigitated metallic templates. Supplementary Fig. S4 illustrates the electrode fabrication. The bicontinuous nickel scaffold for the electrodes was fabricated by electrodepositing nickel through a polystyrene (PS) opal self-assembled on a glass substrate with interdigitated gold templates, and then removing the PS. The interdigitated gold templates for the microbattery electrodes were fabricated by sputtering 8 nm of chromium followed by 70 nm of gold on a 1-mm thick soda lime glass slide. The gold and chromium were then etched into 5–10-mm long interdigitated rectangles, called fingers, connected to two 4-mm wide contact pads such that every other finger was electrically connected and neighbouring fingers were electrically isolated, making the templates for an interdigitated anode and cathode cell. Three templates with different finger area, width and separation ( Supplementary Table S3 ) were used to test the influence of electrode width and spacing on the energy and power density. The glass slide with interdigitated gold templates was then diced into smaller microbattery substrates, piranha cleaned for 10 min, and then immersed in Millipore water with 2.2% by weight 3-mercapto-1-propanesulfonic acid and sodium salt for 3 h and rinsed to prepare them for PS opal growth. The substrates were positioned vertically in a colloid solution of 330- or 500-nm (in diameter) PS spheres and set on a hot plat at 55 °C, covered and left for 24–30 h until the solution was dry. During evaporation, the spheres at the receding water–substrate meniscus are self-assembled onto the substrate into an opal, typically face centred cubic in structure. The substrates were then sintered at 96 °C for either 12 (opal made from 330-nm PS spheres) or 16 h (opal made from 500-nm PS spheres), to increase the interconnect size between the PS spheres. The diameter of the interconnects could be made up to 58% of the pore diameter with sintering and electropolishing [25] . The solution of PS spheres used to fabricate the opals was made by combining 1.2 g of an 8 wt% PS sphere solution with 40 g of Millipore water. The nickel for the anode and cathode 3D scaffold was electrodeposited through the PS opal for about 20 min at a constant −2.0 V versus a nickel reference electrode in commercial plating solution. The nickel grew both vertically and horizontally through the PS opal as it was plated. The typical width and height of the electrodes with template T1 was 33 μm wide and 15 μm tall. The nickel scaffold could be made up to 96.4% porous by maximizing the diameter of the interconnects and electropolishing the nickel after removal of the PS [25] . The PS was removed by immersing the plated substrates in tetrahydrofuran for 5 h followed by oxygen plasma etching at 400 mTorr for 10 min. The resulting nickel structure was a network of interconnecting pores, each pore adjoined by 12 others, which acted as a current collector and provided the scaffold for the microbattery electrodes. In the microbattery cells presented here, the pore size of the nickel scaffold was 500 and 330 nm with 200 and 115 nm diameter interconnects, approximately 87% porous. Anode and cathode electrodeposition The anode and cathode electrolytic materials were sequentially electrodeposited on the nickel scaffold. Voltage-controlled, pulsed electrodeposition was used to ensure conformal coating of the active materials throughout the 3D structure. Supplementary Figure S5 shows the process flow diagram for fabricating the full microbattery cells. A nickel–tin alloy was electrodeposited onto the nickel scaffold corresponding to the anode. MnOOH was then electrodeposited on the nickel scaffold corresponding to the cathode. Supplementary Method contains the plating-solution chemistries and voltage-deposition profiles. Finally, the substrate was immersed in molten lithium salts, LiNO 3 and LiOH, at 300 °C for 30 min to form lithiated manganese oxide. Figure 1b shows cross-section micrographs of the nickel–tin-coated anode and lithiated manganese oxide-coated cathode. The materials were chosen because they could be conformally fabricated in 3D. The thickness of the electrodeposited anode (30–90 nm) and cathode (17–67 nm) layers determine the solid-state ion and electron transport lengths. The volume of active material varies from 14 to 45% of the available electrode volume, depending on the active layer thickness and pore diameter. Figure 1d shows the interdigitated microelectrodes with fully integrated anodes and cathodes. The centre-to-centre distance between electrodes (27–50 μm) governs the ion transport length in the electrolyte. Electrochemical testing of the microbattery The microbattery substrate was covered with TorrSeal after the electrode fabrication, except for the area to be tested. The anode and cathode were independently charged to 0.05 and 4.0 V versus lithium metal in 1:1 ethylene carbonate and dimethyl carbonate with 1 M LiClO 4 liquid electrolyte. The microbattery cell was then capped with a sheet of silicone and tested by galvanostatically discharging the cells from 4 to 2 V at various C rates. At a 1 C rate, the cell discharges in 1 h, and at a C rate of N , the cell discharges at N times the 1 C current. Supplementary Note 2 shows the energy-storage reactions. Microbattery cell characterization The energy and power density of the microbattery cells were obtained by measuring the voltage and current during the cell discharge, calculating the total energy and power, and normalizing the energy and power to the volume of the microbattery cell. During the cell discharge, the time ( t ), voltage ( V ) and current ( i ) were recorded every second or for every 50 mV drop in cell voltage, whichever time is smaller. Each measurement corresponded to a time d t , during which a set number of Coulombs were discharged by the cell, d q = i* d t . The energy discharged at each time was calculated by the product of the voltage and d q . The total microbattery cell energy is the sum of the energy discharged at each d t for the entire discharge time. The power of the microbattery at each time was calculated by the product of the cell voltage and current. The power density values presented are the average power density over the entire discharge. The microbattery cell volume includes the total volume occupied by the electrode (anode, cathode, Ni current collector and electrolyte in the porous 3D electrode) and the electrolyte in the separation between the electrodes. The volume was calculated by multiplying the height of the microbattery cell by the total area of the cell. The height of the microbattery electrodes was correlated with the width of the electrodes and thus could be calculated for the microbattery cell by measuring the average width of the electrodes in the cell. This allowed non-destructive height measurements of the microbattery cells. The ratio of electrode height-to-width was measured on sacrificial electrodes in an SEM. The height-to-width ratio was 0.45 for electrodes made with 500-nm PS spheres and 0.39 for the electrodes made with 330-nm PS spheres. How to cite this article: Pikul, J. H. et al . High-power lithium ion microbatteries from interdigitated three-dimensional bicontinuous nanoporous electrodes. Nat. Commun. 4:1732 doi: 10.1038/ncomms2747 (2013).